Biology of a widespread uncultivated archaeon that contributes to carbon fixation in the subsurface Subsurface microbial life contributes significantly to biogeochemical cycling, yet it remains largely uncharacterized, especially its archaeal members. This 'microbial dark matter' has been explored by recent studies that were, however, mostly based on DNA sequence information only. Here, we use diverse techniques including ultrastuctural analyses to link genomics to biology for the SM1 Euryarchaeon lineage, an uncultivated group of subsurface archaea. Phylogenomic analyses reveal this lineage to belong to a widespread group of archaea that we propose to classify as a new euryarchaeal order (‘ Candidatus Altiarchaeales’). The representative, double-membraned species ‘ Candidatus Altiarchaeum hamiconexum’ has an autotrophic metabolism that uses a not-yet-reported Factor 420 -free reductive acetyl-CoA pathway, confirmed by stable carbon isotopic measurements of archaeal lipids. Our results indicate that this lineage has evolved specific metabolic and structural features like nano-grappling hooks empowering this widely distributed archaeon to predominate anaerobic groundwater, where it may represent an important carbon dioxide sink. Archaea are important players in global biochemical cycles. They can utilize a variety of organic and inorganic electron donors and acceptors and for instance contribute substantially to nitrogen cycling in soil and sea via ammonia oxidation [1] , [2] , [3] . Unique mechanisms for carbon turnover by archaea can lead to production or consumption of methane, an important greenhouse gas, via e.g. anaerobic oxidation of methane [4] , [5] . Archaea have also the ability to assimilate CO 2 by at least three different fixation pathways [6] and are consequently adapted to special microbial niches out-competing their bacterial counterparts [7] . Other than niches, entire biotopes dominated by one single archaeal species are rare, and these archaea have not been studied in the past concerning their metabolic capabilities and contribution to Earth’s biochemical cycles [8] , [9] , [10] , [11] . Although environmental genomics has led to the characterization of many novel archaeal lineages, like ARMAN (archaeal Richmond Mine acidophilic nanoorganisms) [12] , [13] and other members of the DPANN superphylum [14] , there is still a great level of novelty in nature that remains unexplored [15] . These linages often escape regular 16S rRNA gene screenings [12] and may harbor unexpected metabolic diversity and unusual cell structure [12] , [13] , [16] . An example of a genetically unexplored archaeal lineage is represented by the biofilm-forming SM1 Euryarchaeon, which has been described as a model organism for cold-loving archaea [11] . This archaeon was discovered to either live in close association with sulfide-oxidizing bacteria in sulfidic streamlets [17] , [18] or as an almost single species biofilm in oxygen-free subsurface aquifers [9] , [10] , [11] . Similar to ARMAN [12] , the SM1 Euryarchaeon may have escaped regular 16S rRNA gene profiling but was found to be widespread in sulfidic springs in Europe when appropriate 16S rRNA gene primers were used [18] . Novel archaeal lineages have been shown to have unusual biology, as assessed by genomics, cryo-electron tomography and other technologies directly applied to environmental samples [12] , [13] , [16] , [19] . ARMAN for instance, have a highly unexplored genetic repertoire [13] and were one of the first archaea mentioned in the literature showing a double-membrane cell envelope [16] . Metagenomics can nowadays deliver near-complete to complete genomes of uncultivated organisms from environmental samples [20] . This cultivation-independent technology appears very useful for studying microbial life in nature, particularly when coupled to other technologies for inferring structural and genetic information simultaneously [12] , [13] . Here, we integrate metagenomics, metatranscriptomics, focused-ion beam scanning electron microscopy (FIB-SEM), transmission electron microscopy (TEM), Nano Secondary Ion Mass Spectrometry (NanoSIMS), Raman microspectroscopy, analysis of stable carbon isotope composition of lipids, and immunological analyses to investigate genomic, structural and metabolic features of the SM1 Euryarchaeon lineage. Our analysis targeted the Mühlbacher Schwefelquelle (Germany), where previous investigations revealed an SM1 Euryarchaeon member to be the dominant organism in biofilms, washed up from the subsurface [9] , [10] , [11] (hereafter referred to as SM1-MSI for SM1 Euryarchaeon from Mühlbacher Schwefelquelle). Given the similarity and high abundance of a close relative to SM1-MSI from a second subsurface site (Crystal Geyser, USA: SM1-CG), we extended our genomic analysis to this organism. Our results provide genomic, structural and metabolic information for a widespread, novel archaeal lineage, which has the capability to predominate its subsurface biotope by autotrophic growth. Population structure and genomics of SM1-MSI The uncultivated SM1 Euryarchaeon SM1-MSI forms an almost single species biofilm in a cold, sulfidic spring (Mühlbacher Schwefelquelle, close to Regensburg, Germany), which was drilled in 1925 (ref. 10 ). Biofilms are constantly washed up from the subsurface [9] , making them accessible for laboratory experiments. Within biofilms, the coccoid-shaped archaeal cells were spaced fairly regularly ( Fig. 1 ), with each cell linked to 1–7 cells (mostly 6 cells) by a dense web of cell-cell contact filaments. Depending on the amount of surrounding extracellular polymeric substance (EPS), which covered the thin surface structures, the threads appeared occasionally as tubes or bars ( Fig. 1 ). Overall, the cells and threads formed a strongly connected, but spacious and thus penetrable cellular network. 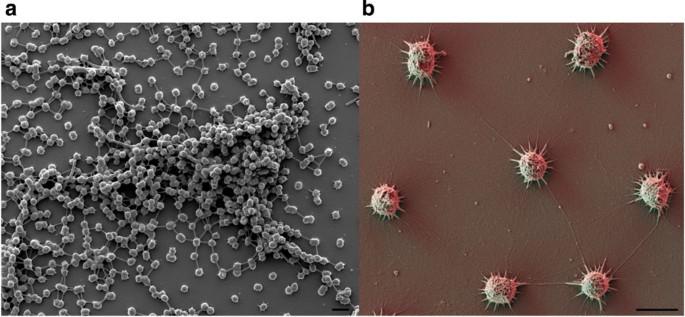Figure 1: Scanning electron microscopy of SM1 euryarchaeal biofilm samples. (a) Overview of the biofilm. Cells are connected by cell surface appendages, which appear like tubes due to the surrounding EPS. Bar: 2 μm. (b) Detailed micrograph of SM1 Euryarchaeon cells showing a typical hexagonal pattern in the biofilm. The cell surface appendages are visible due to the low amount of EPS present. Bar: 1 μm. Figure 1: Scanning electron microscopy of SM1 euryarchaeal biofilm samples. ( a ) Overview of the biofilm. Cells are connected by cell surface appendages, which appear like tubes due to the surrounding EPS. Bar: 2 μm. ( b ) Detailed micrograph of SM1 Euryarchaeon cells showing a typical hexagonal pattern in the biofilm. The cell surface appendages are visible due to the low amount of EPS present. Bar: 1 μm. Full size image The biofilm contained no more than 5% bacteria, mainly sulfate-reducers [11] . Besides SM1-MSI, another archaeon (IM-C4 Euryarchaeon [11] ) was detected at low relative abundances. Cell numbers of IM-C4 were estimated by specific qPCR in nine independent samples to be 0.69±0.67% of all archaeal cells (assuming one 16S rRNA gene per cell). Fluorescence in situ hybridization of IM-C4 confirmed that abundances were so low as to preclude microscopic quantification (<1/100 cells) but revealed a coccoid morphology similar to SM1-MSI ( Supplementary Fig. 1 ). As expected based on 16S rRNA gene profiling [11] , metagenomic shotgun sequencing revealed two archaeal bins, SM1-MSI and IM-C4 ( Supplementary Table 1 ). Relative abundances of these organisms, based on depth of sampling of the reconstructed 16S rRNA gene sequence, were estimated to be 87.7% for SM1-MSI and 1.3% for IM-C4. Bacterial signatures were mainly classified as Deltaproteobacteria, with 3.7% (relative abundance) belonging to Desulfocapsa (phylogenetic tree and relative abundance estimates are depicted in Supplementary Fig. 2 ), supporting results from previous studies [10] , [11] . The genomic bin of SM1-MSI revealed a GC-content of 32.09%, which is in accordance with experimental data [9] ( Supplementary Fig. 3 ). In contrast, SM1-MSI size was 3,333 kbs, a size that greatly exceeds the experimentally determined genome size of 1.5–1.9 Mbps (determined by pulse-field gel electrophoresis as described earlier [21] ). It encoded for 3,294 proteins but most of the single-copy genes were present two or more times, indicating several strains of the SM1 Euryarchaeon in the bin. The analysis of K a K s -ratio (synonymous and non-synonymous mutations) in duplicated single-copy genes revealed a significant difference to randomly mutated genes ( Supplementary Fig. 4 , paired t-test, P -value=0.0004) and provided evidence for the presence of at least two strains in the genomic bin. Consequently, the SM1-MSI bin represents a genomic bin of multiple SM1 euryarchaeal strains thriving in subsurface biofilms. In other words, this genomic bin is a mixture of multiple SM1 euryarchaeal strains, whereas none of the genomes could be closed (many single nucleotide polymorphisms corresponding to strain variation were likely hampering the assembly process). Almost the entire SM1-MSI genome was sampled at least once, since the completeness of the SM1-MSI bin was estimated 98% based on marker genes ( Supplementary Fig. 5 ). From the Mühlbacher Schwefelquelle site, we also recovered 1.374 Mb of genome sequence for IM-C4 (GC-content 48.48%; Supplementary Table 1 and Supplementary Fig. 3 ), which we estimated to represent 90% of the complete genome. Genome reconstruction of SM1-CG from Crystal Geyser Given 16S rRNA gene sequence evidence that a representative of the SM1 Euryarchaeon lineage was abundant in Crystal Geyser water filtration samples (Utah, USA), we also analyzed metagenomic datasets from this site. Crystal Geyser was established in 1935 when a drilling project intersected a CO 2 -rich aquifer in the Navajo sandstone. Periodic eruptions deliver to the surface a sequence of microaerobic and anaerobic, ferrous iron-rich, hydrogen sulfide-bearing, cold (17.5 °C) waters. Shotgun paired short read sequences were derived from samples collected onto 3.0 μm filters and post-3.0 μm samples collected onto 0.2 μm filters [22] . Interestingly, the SM1 Euryarchaeon was the most abundant organism on the 3.0-μm filters (by a factor of 4.2±1.7 for 8 samples) and second most abundant organism on the 0.2-μm filters. Despite multiple attempts using different data subsets and assemblies from different samples, all genomes were quite fragmented; however, genomic data from only one population was assembled, based on analysis of the marker gene inventory. We attribute the fragmentation to strain sequence variation. Contigs were assigned to the SM1 Euryarchaeon lineage based on the combination of high coverage and similarity between predicted protein sequences and previously reported archaeal sequences ( Supplementary Table 1 and Supplementary Fig. 6 ). The assembled fragments encoded ribosomal protein blocks and the 16S rRNA gene sequence, both of which were used for phylogenetic analysis. Based on the fraction of recovered marker genes in the best assembly of SM1-CG, we estimate the genome size to be approximately 1.5 Mbps on the basis of a completeness of 98%. In order to understand the biology of the SM1 Euryarchaeon, we, in the following, linked genomic information of the SM1 Euryarchaeon to intact polar lipid, (ultra)structural, immunological and transcriptomic analyses of the SM1-MSI biofilm. Metabolic predictions from the genomic information were verified/falsified using NanoSIMS and analyzing the stable carbon isotopic composition of archaeal lipids. Unless stated otherwise, the genomic information presented holds true for both genomes, SM1-MSI, from the Mühlbacher Schwefelquelle, and SM1-CG, from Crystal Geyser. The major pathways discussed in this manuscript are summarized in Fig. 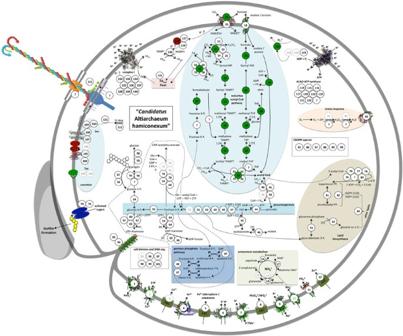Figure 2: Metabolic pathway map of genes encoded in the SM1 euryarchaeal pangenome. Membrane proteins are indicated by symbols or protein structures of subunits (taken from Pfam database). Predicted proteins are indicated by numbers, which can be found inSupplementary Table 2. Grey numbers were found in SM1-MSI but not for SM1-CG. Specific enzymes were tested for presence of corresponding mRNA: Enzymes labeled in green were also detected in the mRNA pool of the biofilm, while enzymes with red color were absent in mRNA pool. Interrogation marks indicate potential metabolic pathway reactions that are likely present but are lacking evidence in the fragmented genomic bins. 2 and corresponding annotations are provided in Supplementary Table 2 . Figure 2: Metabolic pathway map of genes encoded in the SM1 euryarchaeal pangenome. Membrane proteins are indicated by symbols or protein structures of subunits (taken from Pfam database). Predicted proteins are indicated by numbers, which can be found in Supplementary Table 2 . Grey numbers were found in SM1-MSI but not for SM1-CG. Specific enzymes were tested for presence of corresponding mRNA: Enzymes labeled in green were also detected in the mRNA pool of the biofilm, while enzymes with red color were absent in mRNA pool. Interrogation marks indicate potential metabolic pathway reactions that are likely present but are lacking evidence in the fragmented genomic bins. Full size image SM1-MSI features a distinct glycosidic diether lipid profile The high-performance liquid chromatography electrospray ionization mass spectrometry analysis of intact polar lipids (IPLs) in biofilm samples taken from the Mühlbacher Schwefelquelle revealed a dominance of archaeal (94%) versus bacterial lipids (6%; Supplementary Fig. 7 ). The archaeal IPLs consist of core diether lipids with (i) two phytanyl chains (C 20 -C 20 archaeol, AR) and (ii) a combination of one phytanyl and one sesterterpanyl chain (C 20 -C 25 extended archaeol, Ext-AR), which is in accordance with the detection of genes for the synthesis of ether lipids via the mevalonate pathway in the SM1 genomes ( Fig. 2 and Supplementary Table 2 ). Archaeal diethers were composed of monoglycosyl (1G) and diglycosyl (2G) headgroups, and a tentatively identified pentose-hexose headgroup. The major IPLs are 1G-AR and 2G-AR, representing 34 and 57% of total archaeal IPLs ( Supplementary Fig. 7 ). SM1 cells possess double-membranes and nano-grappling hooks The two SM1 Euryarchaeon genomes did not encode genes involved in motility, flagellation or pili production. However, both genomes from the German site (SM1-MSI) and from the US site (SM1-CG) harbor genes for hamus (plural hami) subunits. Hami are specialized cell surface appendages with barb-wire like filamentous structures and nano-grappling hooks at their distal end (diameter approx. 60 nm; Fig. 3a ). These appendages have only been described for SM1 found near Regensburg, Germany [10] , [19] . Genes potentially encoding for the major hamus subunit were identified by searching the predicted proteome with sequence motifs that had been identified in a previous investigation of the hami [19] . The gene sequences did not reveal any homologues in public databases and exhibited the presence of sec signal peptides. Thus, the proteins seem to be secreted via the Sec pathway into the periplasm ( Fig. 2 , Supplementary Table 2 ). 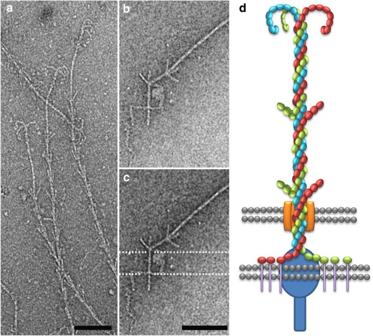Figure 3: Hamus formation, structure and anchorage in SM1 euryarchaeal double membrane. (a) Electron micrograph of hamus filaments (negatively contrasted) as found in the biofilm. Bars: 100 nm. (b,c) Hamus anchoring structure as visualized after release of the hami by dissolving the membrane. Inc, the positions of the two membranes are indicated (white line). (d) Assembly and formation model, based on microscopical and genetic data. The individual threads (colored differently but composed of the same subunits) are formed at the inner membrane, and the hamus structure is built in the periplasm, before being pushed through the outer membrane. The first prickle appears right outside of the cell. Figure 3: Hamus formation, structure and anchorage in SM1 euryarchaeal double membrane. ( a ) Electron micrograph of hamus filaments (negatively contrasted) as found in the biofilm. Bars: 100 nm. ( b , c ) Hamus anchoring structure as visualized after release of the hami by dissolving the membrane. In c , the positions of the two membranes are indicated (white line). ( d ) Assembly and formation model, based on microscopical and genetic data. The individual threads (colored differently but composed of the same subunits) are formed at the inner membrane, and the hamus structure is built in the periplasm, before being pushed through the outer membrane. The first prickle appears right outside of the cell. Full size image The anchoring of the hami in SM1-MSI archaea was assessed by different electron microscopy-based techniques. Thin sectioning and preliminary electron tomographic analysis revealed that they are most likely anchored within the cell wall, the cytoplasm and perhaps even in an additional basal structure within the cytoplasm. The cell wall of the SM1 Euryarchaeon consists of an outer membrane that is separated from the cytoplasmic membrane by periplasmic space of about 30 nm ( Fig. 4 ). No peptidoglycan- or pseudopeptidoglycan-layer was identified in ultrastructural analysis, nor any associated biosynthesis proteins were detected in the genomes. Thin sections of the cells further revealed the presence of a thick extracellular polymeric substance (EPS-)layer and hami forming a dense network around cells. Hami were anchored in both membranes, with a protrusion into the cytoplasm (‘thorn’, model in Fig. 3b,c ). Based on electron microscopic analysis of membrane-released hami, we propose a model for the assembly of the hamus structure ( Fig. 3d ), which represents a convergent evolution to type IV pili formation in bacteria, involving the outer membrane [23] . In addition, other, so far unidentified proteins appeared to be involved in hamus structure assembly as observed in Fig. 3 (e.g. outer membrane channel, thorn). 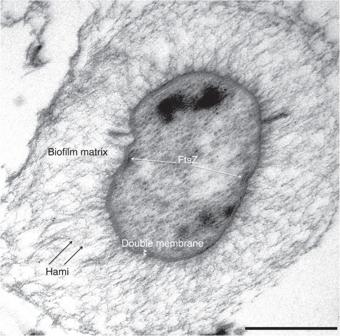Figure 4: Electron micrograph (ultrathin section) of a SM1 euryarchaeal cell in the biofilm after high-pressure freezing. The cell is surrounded by an EPS matrix and cell surface appendages (hami), which go beyond the matrix. The cell has two membranes with a faint periplasm. FtsZ aggregates (Fig. 5) are located at the inner membrane. Bar: 500 nm. Figure 4: Electron micrograph (ultrathin section) of a SM1 euryarchaeal cell in the biofilm after high-pressure freezing. The cell is surrounded by an EPS matrix and cell surface appendages (hami), which go beyond the matrix. The cell has two membranes with a faint periplasm. FtsZ aggregates ( Fig. 5 ) are located at the inner membrane. Bar: 500 nm. Full size image Of several identified genes involved in cell division ( Fig. 2 ) the FtsZ gene was of special interest as FtsZ proteins are constantly present but only aggregated when cells divide [24] . TEM and FIB-SEM images of SM1-MSI biofilm cells revealed the presence of FtsZ-resembling, electron-dense rings in the cytoplasm underneath the cell membrane, which were co-localized to invagination sites of dividing cells ( Fig. 5 ). In subsequent immuno-staining experiments with antibodies against FtsZ homologs, SM1 Euryarchaeon cells were shown to indeed accumulate FtsZ between separating cells ( Fig. 5c–e ). Since nearly all cells reconstructed using FIB-SEM were observed to possess these rings ( Fig. 5b ), it is assumed that SM1 euryarchaeal cells in biofilm samples were under active division when harvested. This finding was confirmed via nucleic acid staining (using DAPI and fluorescence microscopy), revealing that ~73% of SM1-MSI cells in biofilms (2500 cells counted) were undergoing cell division. In addition, SM1 population revealed a high viability with ~95% of all SM1-MSI cells being alive at the time of sampling [9] . 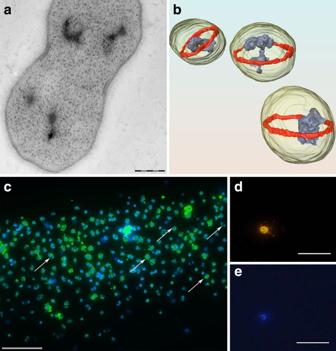Figure 5: FtsZ and its localization in SM1 euryarchaeal cells indicating a continuous division of cells in the subsurface biotope. (a) Thin section of a dividing SM1 cell. An electron-dense zone is observed beneath the cytoplasmic membrane at the invagination. Bar: 200 nm. (b) Three-dimensional reconstruction (FIB-SEM) of SM1 cells in the biofilm. Electron-dense parts are labeled in red, precipitates of unknown chemical composition are in grey, cells walls are shown in brown. (c) Fluorescence micrograph of a biofilm sample showing DNA in blue (DAPI) and FtsZ (labeled with FtsZ antibody) in green. FtsZ is located in the septum area of dividing cells. Bar: 10 μm. (d) Single SM1 Euryarchaeon cell, labeled with anti-FtsZ (green) and anti-hamus (orange) antibodies showing that FtsZ is expressed in SM1 Euryarchaeon cells. Bar: 5 μm. (e) Same micrograph as in D but DAPI staining is indicated in blue. Bar: 5 μm. Figure 5: FtsZ and its localization in SM1 euryarchaeal cells indicating a continuous division of cells in the subsurface biotope. ( a ) Thin section of a dividing SM1 cell. An electron-dense zone is observed beneath the cytoplasmic membrane at the invagination. Bar: 200 nm. ( b ) Three-dimensional reconstruction (FIB-SEM) of SM1 cells in the biofilm. Electron-dense parts are labeled in red, precipitates of unknown chemical composition are in grey, cells walls are shown in brown. ( c ) Fluorescence micrograph of a biofilm sample showing DNA in blue (DAPI) and FtsZ (labeled with FtsZ antibody) in green. FtsZ is located in the septum area of dividing cells. Bar: 10 μm. ( d ) Single SM1 Euryarchaeon cell, labeled with anti-FtsZ (green) and anti-hamus (orange) antibodies showing that FtsZ is expressed in SM1 Euryarchaeon cells. Bar: 5 μm. ( e ) Same micrograph as in D but DAPI staining is indicated in blue. Bar: 5 μm. Full size image Consequently, one can assume that biofilm pieces sampled at the MSI site are rather from a continuously growing subsurface biofilm than from a static system. This continuous growth of the archaea coupled to a very low but natural statistical error rate in replicating genomes [25] may result in a heterogeneous genome composition of SM1 strains. This natural strain variation may have complicated genome recovery as mentioned above. SM1 has a novel type of archaeal reductive acetyl-CoA pathway Since the Mühlbacher sulfide spring water from where SM1-MSI Euryarchaeon was sampled is poor in organic substances (dissolved organic carbon at MSI site 1.3 mg/l on average), it is not surprising that genes for the transport and assimilation of complex organic compounds, amino acids and sugars were not identified in SM1 genomes ( Fig. 2 , for details on transporter and ammonia assimilation see Supplementary Note 1 ). Moreover, the SM1 genomes did not encode for β-oxidation enzymes, electron transferring flavoproteins, acyl-CoA dehydrogenases, crotonases, enzymes involved in fermentation or carbohydrate-metabolizing enzymes. Tricarboxylic acid (TCA) cycle and the glyoxylate cycle were incomplete. Instead, we inferred from the genomic and transcriptomic data that the SM1 anabolism centers around activated acetic acid, acetyl-CoA, which appears to be a starting point of the biosynthesis of cellular building blocks ( Fig. 2 ). The presence of an unidirectional gluconeogenetic fructose-1,6-bisphosphate aldolase/phosphatase [26] suggests that the metabolic fluxes are oriented from acetyl-CoA to phosphoenolpyruvate (via ferredoxin-dependent pyruvate synthase and phosphoenolpyruvate synthase) and further to fructose-6-phosphate ( Fig. 2 ; for biosynthetic reactions see next paragraph). The SM1 genomes contain a homolog of AMP- and pyrophosphate-forming acetyl-CoA synthetase. This is the only enzyme encoded in the SM1 genome that is responsible for the activation of a carboxylic acid. Neither genes for ADP-forming synthetases (including the TCA cycle enzyme succinyl-CoA synthetase) nor CoA-transferase and phosphotransacetylase/acetate kinase homolog were identified. Pyrophosphate formed in the acetyl-CoA synthetase reaction could only be hydrolyzed by a soluble pyrophosphatase as genes for a membrane-bound pyrophosphatases are missing. Therefore, an activation of acetate is hypothesized to be accompanied by a conversion of ATP into AMP and two phosphates, i.e. by a hydrolysis of two high-energy bonds of ATP making the reaction irreversible. The gene for this putative acetyl-CoA synthetase is located next to a gene encoding a major facilitator superfamily transporter with the similarity to a formate/oxalate antiporter. This protein might be involved in acetate uptake, possibly linked to formate antiport. Although transcription was shown for the putative acetyl-CoA synthase in SM1-MSI biofilms, labeling experiments of the SM1-MSI cells using U- 13 C-labeled acetate (80 μM) and NanoSIMS did not show assimilation of 13 C isotopes in SM1 archaeal cells after one day and after three days of incubation time, respectively. Moreover, the spring water did not contain any measurable amount of acetate (detection limit 5 μM). From the current perspective of the data, anabolism of SM1 based on acetate uptake appears unlikely. SM1 genomes possess genes for the archaeal version of the reductive acetyl-CoA (Wood-Ljungdahl) pathway ( Fig. 2 ) without enzymes encoding for methanogenesis (mcr and biosynthesis pathways for CoM and CoB). As in the reductive acetyl-CoA pathway of methanogenic archaea, the SM1 pathway makes use of methanofuran and tetrahydromethanopterin (THMPT) as the C 1 -carriers. However, some of these enzymes showed atypical traits compared to those previously described in archaea [6] . In SM1, the archaeal factor 420-dependent THMPT dehydrogenase is replaced by a NAD(P)-dependent enzyme of potential bacterial origin, known mainly from methylotrophic bacteria [27] and thus likely acquired via HGT (the other identified genes, including the key enzyme CO dehydrogenase/acetyl-CoA synthase, are of archaeal origin; Supplementary Table 3 ). Furthermore, genes for the biosynthesis of factor 420 (F 420 ) were not identified, and the presence of F 420 could not be detected in the SM1 Euryarchaeon cells from a different site [28] . For the reduction of methylene-THMPT, NAD(P)-dependent enzymes have not been detected, but we suggest that a putative methylene-THF reductase which is similar to a still unidentified enzyme from ANME genome [29] may be responsible for the compensation of this reaction in SM1. In comparison, other archaea with reductive acetyl-CoA pathway (like methanogens) utilize F 420 H 2 in methylene-THMPT-dehydrogenase and methylene-THMPT-reductase reactions. The ‘classical version’ of the reductive acetyl-CoA pathway is fully reversible and can function for both acetyl-CoA synthesis and oxidation [30] . Although the redox potential of NAD(P) + /NAD(P)H (−320 mV) compared to F 420 /F 420 H 2 (−360 mV) would favor acetyl-CoA catabolism rather than autotrophic CO 2 fixation in SM1, stable carbon isotope analysis of SM1-MSI lipids revealed relatively 13 C-depleted core AR (δ 13 C=–71‰). Interestingly, although the detected lipid profile of SM1 is neither congruent with those from methanogens [31] or ANME [32] , the co-occurrence of 13 C-depleted archaeal and bacterial lipids (mono- and diether lipids ranged from –30‰ to –70‰) has been only reported in methane seep sediments [33] . For comparison, we additionally obtained stable carbon isotopic values of CO 2 (–18‰) and CH 4 (–63‰) sampled from groundwater ( n =3 samples). In sum, given the absence of measurable acetate concentrations and the above-mentioned δ 13 C values of CO 2 at –18‰ in the groundwater from the Mühlbacher Schwefelquelle, these observations coupled to the genomic information suggest carbon dioxide fixation by SM1 cells using the Wood-Ljungdahl pathway. The functioning of the reductive acetyl-CoA pathway requires strictly anaerobic conditions. The SM1 cells grow in flowing oxygen-depleted groundwater (Germany) and stratified highly suboxic/anaerobic groundwater (USA) [11] , [18] . Presence of hydrogen sulfide in both systems may support strictly anaerobic metabolism. In case of fluctuating oxygen concentrations in groundwater, the SM1-MSI encodes rubrerythrin and associated oxygen stress response enzymes ( Fig. 2 ). Overall, we conclude that the major anabolic reactions performed by the SM1 Euryarchaeon are assimilation of carbon dioxide into activated acetic acid using a novel variant of the reductive acetyl-CoA pathway, whose enzymes were transcribed in vivo ( Fig. 2 ). Biosynthetic reactions in SM1 Euryarchaeon Pentose phosphates are synthesized in SM1 Euryarchaeon either through a reversed ribulose monophosphate pathway or via transketolase and transaldolase reactions ( Fig. 2 ). Formaldehyde synthesized in the hexulose-6-phosphate synthase reaction of the ribulose monophosphate pathway may be scavenged in spontaneous reaction with THMPT or tetrahydrofolate (THF) or through oxidation with one of the aldehyde dehydrogenases present in SM1 genomes. Apart from the genes for THMPT-dependent enzymes, SM1 genome encodes several THF-dependent enzymes, which are transcribed in the biofilm samples. The corresponding enzymes probably provide C 1 -units for purine biosynthesis, as in case of Methanosarcina barkeri [34] . Synthesis of glutamate precursor 2-oxoglutarate proceeds probably through re -citrate synthase, aconitase and isocitrate dehydrogenase. These biosynthetic reactions represent the core of nucleotide and aminoacid biosynthesis in the SM1. Gluconeogenesis products glucose-6-phosphate and fructose-6-phosphate are used for synthesis of a variety of activated forms of sugars, like rhamnose, mannose, fucose and acetylmuraninate. These sugars could serve as substrates for the many glycosyltransferases (44 in total) found in the genome and/or result in synthesis of biofilm polymers ( Fig. 4 ), which was shown to be mainly comprised of carbohydrates [9] . Noteworthy, glucose-6-phosphate is also a precursor for the storage product glycogen, which is a great resource for activated sugars for biofilm synthesis. Indeed, using Raman microspectroscopy, accumulation of glycogen in most SM1 Euryarchaeal cells was demonstrated ( Supplementary Fig. 8 ). Glycogen can afterwards be either degraded by an amylase or a phosphorylase homolog. Since SM1 bins do not code for a potential hexokinase, degradation of glycogen via amylase appears to be a metabolic impasse. Phosphorolytic cleavage of glycogen is more reasonable than hydrolytic cleavage, even though phosphorylases encoded in the SM1 genome have only low similarity with characterized ones ( Fig. 2 ). In sum, the SM1 Euryarchaeon appears to have a well-equipped sugar biosynthesis machinery, which enables biofilm formation—a potentially essential adaptation to dominate subsurface biotopes at the Mühlbacher Schwefelquelle and other sulfur springs. SM1 energy metabolism remains encoded in genetic dark matter No genes in the SM1 genomes could be clearly matched to enzymes that may be conclusive of potential electron donors or acceptors. We identified neither membrane-bound enzymes transferring electrons (to e.g. nitrate or nitrate) nor homologues of cytochromes. However, some information regarding proton gradient establishment and energy conservation could be inferred from the genomic data acquired. CO (present in essentially all groundwater ecosystems [35] ) or H 2 could be a potential electron donors for SM1 Euryarchaeon growth resulting in reduced ferredoxin (see below). Concerning H 2 , the SM1 genomes do, however, not have genes encoding hydrogenases, just like the ANME-1 genome [36] . Although homologues of the electron shuttling [NiFe]-hydrogenase subunits were encoded and transcribed in SM1-MSI ( Fig. 2 ), neither catalytic subunits of [NiFe]-hydrogenase nor any [FeFe]-hydrogenases were identified. Nevertheless, genes for hydrogenase maturation enzymes like HypA, which help to incorporate nickel [37] , were present in the SM1-MSI genomes. These enzymes might also be involved in the maturation of CO-dehydrogenase/acetyl-CoA synthase. Another source of reduced ferredoxin could be electron bifurcation [38] . The presence in SM1-MSI genome of homologues of heterodisulfide reductase genes (of a bacterial origin) located next to a gene for a putative ferredoxin:NADPH oxidoreductase suggests a potential electron transfer from NADPH to ferredoxin. However, these genes (e.g., the subunit B of heterodisulfide reductase gene in Fig. 2 ) were not present in SM1-CG and were not expressed in the biofilm samples (SM1-MSI). Consequently, these potential electron bifurcation reactions may not be essential for SM1 Euryarchaeon to proliferate in its biotope and rather present a potential adaptation under different growth conditions. Reduced ferredoxin might be used for the generation of the proton gradient mediated by a Complex 1-like oxidoreductase ( Fig. 2 ). The genes of this complex (missing the NADH-binding module) have been reported in genomes of subsurface bacteria [39] and are hypothesized to function with ferredoxin [40] . The proton gradient can then be utilized by ATP-synthase complex for the generation of ATP. In addition, formate in the periplasmic space might be oxidized by a membrane-bound formate dehydrogenase present in the SM1 genomes. As its catalytic site appears to face the periplasm, this would lead to the liberation of two protons and formation of a proton gradient enabeling ATP synthesis as mentioned above. It is tempting to believe that the cell surface appendages (hami) of SM1, whose genes are encoded next to metabolic genes (CO dehydrogenase/acetyl-CoA synthase), may be involved in electron transport. Outside the cells, potential electron acceptors could be e.g. ferrous iron, an abundant constituent of the Crystal Geyser water (as it was shown by Geobacter sulfurreducens [41] ). Alternatively, electrons could be passed to other microorganisms such as the sulfate-reducing bacteria that are closely associated with SM1-MSI [11] . However, preliminary experiments with SM1 biofilms from the German site did not show an increased conductivity of the microbial biofilm compared to the spring water ( Supplementary Fig. 9 ). Consequently, electron uptake or release via the biofilm matrix and the cell surface appendages appeared to be unlikely. ANME-1 is the lineage with the greatest number of similar protein sequences compared to SM1-MSI (13% of all proteins, Supplementary Fig. 10 ). Comparisons to the ANME lineage metabolic characteristics may provide clues to as yet unresolved parts of the SM1 metabolism. For example, with regard to dissimilatory or assimilatory sulfate reduction, only a homologue of the adenylyl sulfate kinase was found. In this respect, SM1 Euryarchaea are similar to anaerobic methanotrophic archaea of the ANME-1 group. More importantly, anaerobic methanotrophs of ANME-2 group are capable of sulfate reduction to zero-valent sulphur compounds via an unknown mechanism [42] . Nevertheless, in contrast to ANME-2 cells [42] , zero-valent sulfur could not be detected in Raman spectra of SM1-MSI cells ( Supplementary Fig. 8 ) providing no support for SM1 performing a non-thermophilic sulfate reduction. Although function prediction of genes may raise speculation about formate, carbon monoxide or hydrogen as electron donors, the entire electron transport chain remain hidden as genetic dark matter in the sequence information provided herein. The oxidation of ferredoxin appeared to be central for SM1 in establishing a proton gradient for energy conservation, while fermentation could be ruled out. SM1 represents a novel and diverse lineage of Euryarchaeota The lineage represented by the SM1 Euryarchaeon was so far only defined by environmental 16S rRNA gene sequences and suspected to be methanogenic [8] . The availability of genomic data for two representatives of the SM1 Euryarchaeon lineage from two sites and one relative, IM-C4, now enabled us to investigate their placement in the archaeal phylogeny by using multiple protein markers. Bayesian phylogenetic analysis of 56 concatenated ribosomal proteins from 142 archaeal genomes indicated that SM1-MSI, SM1-CG and IM-C4 form a robust monophyletic cluster laying on a long branch sister to the Methanococcales ( Fig. 6 ). However, their placement was unstable, as observed for very fast evolving nano-sized lineages with few available close relatives such as the ARMAN or Nanoarchaeota, whose clustering may not reflect true evolutionary relationship [43] , [30] . Noteworthy, the availability of the deep branching IM-C4 representative likely helped avoiding a well-known tree reconstruction artifact by breaking the long branch leading to the SM1-MSI/CG strains ( Fig. 6 ). We nevertheless applied a number of strategies known to alleviate potential tree reconstruction artifacts such as varying taxonomic sampling, recoding strategies, and use of alternative markers ( Supplementary Fig. 11 and Supplementary Fig. 12 ). In all of these analyses the SM1 Euryarchaeon lineage consistently branched within Euryarchaeota and displayed, apart from a sister relationship to Methanococcales, only two alternative and early branching placements (shown in Fig. 6 ). These results, and the lack of a close relationship to a particular archaeal lineage are also consistent with a specific profile of DNA replication components ( Supplementary Fig. 13 ), including the presence/absence pattern of a few markers that have been recently shown to provide phylogenetic information [44] . The distinctiveness of the SM1 Euryarchaeon lineage and its phylogenetic placement around a few deep euryarchaeal nodes was also confirmed by similarity analysis of the whole proteome predicted for SM1-MSI. In fact, the taxonomic distribution of the closest hits showed a clear dominance of Euryarchaeota, and in particular methanogens, with an enrichment of top hits to the uncultured ANME-1 representative (13% of all proteins, Supplementary Fig. 10 ). 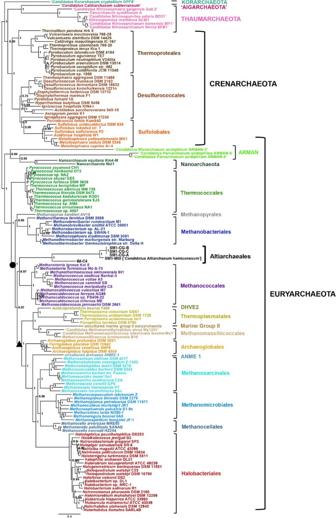Figure 6: Bayesian phylogeny based on 56 concatenated ribosomal proteins (for details see Results andSupplementary Methods). The SM1-MSI, IM-C4 and MSI-CG (A/B/C) represent a distinct euryarchaeal lineage possibly related to Methanococcales. Numbers at nodes indicate posterior probabilities. The scale bar displays the average number of substitutions per site. Two alternative placements for the SM1 lineage are indicated: one obtained by Dayhoff6 recoding of the r-protein dataset (circle), and one from concatenation of 10 universal markers (triangle; seeSupplementary Figs 11 and 12). Figure 6: Bayesian phylogeny based on 56 concatenated ribosomal proteins (for details see Results and Supplementary Methods ). The SM1-MSI, IM-C4 and MSI-CG (A/B/C) represent a distinct euryarchaeal lineage possibly related to Methanococcales. Numbers at nodes indicate posterior probabilities. The scale bar displays the average number of substitutions per site. Two alternative placements for the SM1 lineage are indicated: one obtained by Dayhoff6 recoding of the r-protein dataset (circle), and one from concatenation of 10 universal markers (triangle; see Supplementary Figs 11 and 12 ). Full size image Interestingly, we estimated that a large proportion of the SM1-MSI genes might have been acquired via horizontal gene transfer from bacteria ( Supplementary Fig. 14 ). For 2411 protein sequences, maximum likelihood trees were calculated with potential homologous sequences detected in the NCBI non-redundant database (nr). 851 of these showed branching within bacterial sequences only, indicating that ~25.8% of genes have been potentially acquired via horizontal gene transfer, a similar percentage as reported for haloarchaea [45] . 16S rRNA gene analyses indicated that SM1-MSI, SM1-CG and IM-C4 are representatives of a widespread and diverse archaeal lineage. The SM1 Euryarchaeon lineage clusters phylogenetically with environmental 16S rRNA gene sequences from other cold sulfidic springs close to the Mühlbacher Schwefelquelle (with 100% 16S rRNA gene identity [18] ) and with SM1-CG (~98% 16S rRNA gene identity) from the above mentioned, CO 2 -driven, cold-water geyser (Crystal Geyser). More distant relatives of SM1-MSI (13% difference in 16S rRNA gene sequence) were detected in hot springs (58.5 °C) in the USA, described to be rich in hydrogen [8] , and in Bulgarian hot springs [46] (79 °C; 11% difference in 16S rRNA gene sequence), as well as in ponds and deep-sea environments ( Fig. 7 ). The 16S rRNA gene sequence of the IM-C4 Euryarchaeon places this organism with sequences from archaea from deep-sea sediments, hot springs, aquifers, freshwater ponds and plant reservoirs, branching with SM1-MSI (75.9% 16S rRNA gene identity; Fig. 7 ). 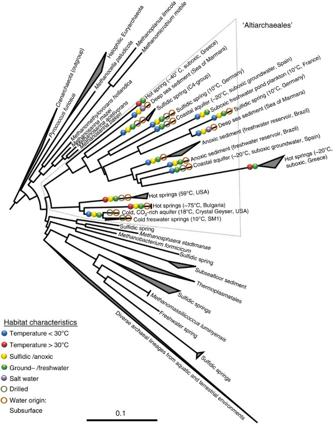Figure 7: Distribution and diversity of SM1-related organisms. The phylogenetic tree is based on 16S rRNA gene sequences from various studies (for accession numbers please seeSupplementary Table 4). The SM1 Euryarchaeon is the representative of a novel archaeal candidate order termed ‘Altiarchaeales’ (frame). Figure 7: Distribution and diversity of SM1-related organisms. The phylogenetic tree is based on 16S rRNA gene sequences from various studies (for accession numbers please see Supplementary Table 4 ). The SM1 Euryarchaeon is the representative of a novel archaeal candidate order termed ‘Altiarchaeales’ (frame). Full size image Altogether, our phylogenetic analyses indicate that the SM1-MSI and SM1-CG are representatives of a new euryarchaeal order-level lineage of anaerobic, aquatic subsurface archaea, for which we propose the candidatus name ‘Altiarchaeales’ (candidatus family ‘Altiarchaeaceae’) indicating their origin in the subsurface (see below for full description). Description of ‘ Candidatus Altiarchaeum hamiconexum’ We here propose the name ‘ Candidatus Altiarchaeum hamiconexum sp. nov.’ for the SM1 Euryarchaeon representatives from the Mühlbacher Schwefelquelle, Sippenauer Moor (main spring) and Crystal Geyser. [Altiarchaeum gen. nov. (Al.ti.archae'um. L. adj. altus, high, deep; N.L. neutr. n. archaeum, a taxonomic unit; N.L. neutr. n. Altiarchaeum, an Archaeum from the deep.] [A. hamiconexum spec. nov. (ha.mi.con.ex'um. L. n. hamum, a hook; L. part. adj. conexus, connected; N.L. neutr. adj. hamiconexum connected by a hook).] Biofilm-forming small coccoid cells (0.4–0.7 μm in diameter) with double membrane. Non-motile. Formation of highly structured cell surface appendages (hami) and extracellular polymeric substances (EPS). Lipids are mainly mono- or diglycosyl diether with two phytanyl chains (C 20 -C 20 ) and a combination of one phytanyl chain and one sesterterpanyl chain (C 20 -C 25 ). The biofilms originate in the deep subsurface of anoxic freshwater springs. In the surface water of sulfidic springs, ‘ Candidatus Altiarchaeum hamiconexum’ forms specific microbial communities together with sulfide-oxidizing bacteria (string-of-pearls community) [18] . Cell division is based on FtsZ. Non-methanogenic, grows on carbon dioxide and potentially also on acetate, formate or carbon monoxide. We also propose the candidatus order ‘Altiarchaeales’ (order nov.), and the candidatus family ‘Altiarchaeaceae’ (fam. nov.). Recent studies have revealed that the subsurface can harbor lineages of microbial life that are vastly unexplored [20] , [39] . Our study expanded knowledge of subsurface biology through genomic and ecophysiological description of a novel archaeal lineage, ‘ Candidatus Altiarchaeum hamiconexum’. This organism is a member of an archaeal clade previously only represented by environmental 16S rRNA gene sequences that were suspected to derive from methanogenic archaea without any other metabolic or genomic evidence [8] . The data presented herein enabled the exclusion of methanogenesis for this lineage. We infer an autotrophic metabolism, in which carbon dioxide fixation is taking place using a novel variant of the archaeal acetyl-CoA pathway. Biofilm formation by the Mühlbacher Schwefelquelle archaea, mediated by (sugar-) polymers and hami, may confer major advantages over other organisms. The biofilm could act as a filter for substrates released into the subsurface water by other microbial community members or, potentially, play a role in electron transfer. Windows into the Earth’s deeper subsurface regions are rare. Analysis of samples collected via contemporary drilling projects is greatly complicated by contamination introduced during drilling. The two spring systems studied here, both established over 75 years ago, regularly discharge large volumes of aquifer fluids sourced dozens to hundreds of meters below ground. Strains of the ‘ Candidatus Altiarchaeum hamiconexum’, adapted to anaerobic environments, are dominant primary producers both of these ecosystems. Such dominance, not observed for any other archaeal lineage, may be common in other deep aquifer systems, where these archaea potentially represent an important sink of carbon dioxide. Sampling, DNA extraction, quality control for shotgun sequencing Samples were taken from the sulfidic spring called Mühlbacher Schwefelquelle, Isling (MSI), near Regensburg (coordinates: 48.98 N, 12.13 E) at a depth of 1 m through a time period of four months [11] . A two-side opened Schott flask allowing a continuous flow through of spring water (approximately 5,500 l h −1 ) was used to filter biofilm droplets with a polyethylene net [11] . Samples were transported to the laboratory on ice, concentrated via centrifugation (10 min, 13,800 × g ) and stored at −80 °C. Metagenomic DNA was extracted using MoBio Power Biofilm DNA kit (MoBio, Carlsbad, USA). Quality with regard to length of metagenomic DNA was verified using agarose gel electrophoresis and the quantity of archaea and bacteria in the samples was determined via qPCR according to established protocols [11] . In brief, 16S rRNA gene copy numbers in 1 μl of metagenomic DNA are amplified using universal and domain-biased primers. For metagenomic library construction, DNA was subjected to paired-end sequencing at LGC Genomics, Berlin (Germany). Using two independent sequencing platforms, Illumina HiSeq 2000 and Roche 454 FLX Titanium, 426,869,764 (average length: 100 bases, approximate insert size: 300 bases) and 246,234 reads (average length 342 bases, approximate insert size: 2750±500 bases) were generated, respectively (LGC Genomics, Berlin, Germany). For the Illumina reads LGC Genomics carried out clipping of sequencing adapters, quality filtering (removal of reads containing Ns, trimming of reads at 3′-end to get a minimum average Phred quality score of 10 over a window of 10 bases and discarding reads shorter than 5 nt using CASAVA tool 1.8.2; http://support.illumina.com/sequencing/sequencing_software/casava.ilmn ) and filtering for paired reads. A subsequent quality check of the LGC Genomics filtered Illumina reads using FASTQC ( http://www.bioinformatics.babraham.ac.uk/projects/fastqc ) showed that no additional filtering was necessary. For 454 reads the program sff_extract.py ( http://bioinf.comav.upv.es/sff_extract ) was used to convert the raw SFF-files to fastq format and clip ends with low quality or adaptor sequences. Reconstruction of 16S rRNA genes and abundance estimation in MSI samples This was performed as described in the Supplementary Methods . Binning and completeness estimation of genomes from MSI site The filtered Illumina paired-end reads were digitally normalized to a maximal k-mer coverage of 130 and a minimal k-mer coverage of 3, resulting in a total of 54,853,038 paired reads [47] . A 10% subset of the normalized reads together with the entire set of 454 paired-end reads was used for a hybrid assembly with MIRA [48] (for details, please see Supplementary Table 1 ; a comparison with other assembly strategies is summarized in Supplementary Table 4 ). Resulting contigs were filtered by a minimal average coverage cutoff of 10 and a minimal length cutoff of 3 kpbs. These quality cutoffs have been shown to be very conservative in order to avoid chimeric sequences in datasets [49] . In addition, the sequenced reads were mapped back to the SM1-MSI contigs. Filtered contigs were manually inspected for large deviations in the coverage distribution that might indicate chimeras. 22 contigs showed large deviations and were checked for proper read-pairing using Tablet ( http://ics.hutton.ac.uk/tablet ). Read-pairing in these contigs did not support chimera assumption, therefore, the contigs were retained. All contigs were searched against a custom set of marker genes from the eggNOG database [50] and blast [51] results were phylogenetically analyzed using MEGAN4 (ref. 52 ) (best hit, bit score cutoff 150). Contigs classified as archaeal were extracted and archaeal bins were further constrained based on GC-coverage plots [53] and phylogenetic placement of the marker genes, i.e. 16S rRNA and hamus subunit genes, which were identified using blastn [51] . These bins were used as custom training sets for Phymm and the PhymmBL algorithm was used for taxonomic classification of the complete assembly [54] . This re-classification of the metagenome expanded the bins by recruiting further contigs based on nucleotide composition. Preliminary annotation of genomes and completeness estimation are described in the Supplementary Methods . Annotation of SM1-MSI genome The SM1-MSI bin was re-annotated using the synteny-supported annotation platform MaGe [55] , [56] . Specific tools that supported the manual annotation and curation are provided in the Supplementary Methods . Sampling, assembly, annotation, binning of CG data Crystal Geyser is located on the east bank of the Green River, 6 km south of the town of Green River, Utah, USA (38° 56.3' N, 110° 8.1' W). 65 L of geyser water was collected as it erupted on November 6th and 8th, 2009. Water samples for metagenomics were filtered sequentially through 3.0 and 0.2 μm polyethersulfone filters (Pall Corporation, NY, USA) via a peristaltic pump, and filters were immediately frozen on dry ice in the field and then stored at −80°C in the laboratory until processing. DNA was extracted via the PowerMax Soil DNA Isolation Kit (MO BIO Laboratories, Inc., Carlsbad, CA). For sequencing, separate 500-bps insert-size libraries were constructed from DNA extracted from the 3.0 and 0.2 μm samples. For the analyses described here, we used sequencing information from nine 3 μm filters, labeled A through J (analysis of the 0.2 μm data and other aspects of the community composition will be reported elsewhere). These filters were essentially replicates, collected from subsamples of the water from the two eruptions. Libraries were sequenced on the Illumina HiSeq platform and resulted in 36 Gb of paired-end sequence (239,247,978 reads at 150 bp per read). Reads were trimmed for quality (using Sickle; Sickle: A sliding-window, adaptive, quality-based trimming tool for FastQ files (Version 1.21), available at https://github.com/najoshi/sickle ) and assembled using the IDBA_UD assembly software [57] using default parameters. Genes were predicted with Prodigal [58] on all contigs >5 kb, using the ‘meta’ option. Predicted proteins on each contig were assigned a preliminary functional annotation based on best blast hits to the UniRef90 database [59] . Because the SM1-CG genome was substantially more highly sampled than any other genome in the 3 μm samples, binning of the genome could be established using coverage and GC content. Multiple assemblies of data subsets were carried out to attempt to improve the genome quality by lowering the coverage, but this conferred no advantage. The best assembled genome came from sample I, and this was used for comparative genomic analysis with SM1-MSI genome. Here, blastp [51] was used to search for protein similarities between the genomes (e-value=10 −5 ) and annotations were only considered if both analyses pathways (for SM1-MSI and SM1-CG) produced identical functional predictions. We compared the representation of SM1-CG in samples A through I by evaluating coverage of scaffolds carrying ribosomal protein S3 (rpS3) genes (the three most abundant organisms in each sample were identical and at comparable relative coverage levels). The rpS3 sequences of SM1 from the samples were identical so only sequences from samples A, B and C were included in our phylogenomic analyses. The SM1-MSI genome (scaffold and protein sequences) is available as Supplementary Data 1 and 2 . Phylogenomic analysis and estimation of horizontal gene transfer These are described in the Supplementary Methods . Transcriptomics of certain metabolic pathways in SM1-MSI For genes for certain key enzymes or for single subunits thereof, transcription was tested via specific mRNA detection in biofilm samples ( Supplementary Table 5 containing list of genes and primers). Total RNA was isolated using the PowerBiofilm RNA Isolation Kit (Mobio Laboratories Inc., Carlsbad, USA) according to manufacturers’ instructions (DNA digestion was performed for 30 min). After precipitation of nucleic acids DNAse treatment was repeated, followed by subsequent reverse-transcription to cDNA (QuantiTect Rev. Transcription Kit, Qiagen, Hilden, Germany). Specific primers were designed using the web tool Primr3v.0.4.0 ( http://biotools.umassmed.edu/bioapps/primer3_www.cgi ; parameters: product size: optimum 400 bp, GC% 40–60%, annealing temperature: 60 °C optimum). Specificity of primers was tested using blast [51] against NCBI NR and the metagenome. CDNA was used for amplification with designed primer pairs individually (denaturation time: 5 min 95 °C; 30 cycles: 45 s 94 °C, 45 s 60 °C, 90 s 72 °C; final elongation: 10 min 72 °C). Positive PCR products were purified (HiYield® Gel/PCR DNA Fragments Extraction Kit; Süd-Laborbedarf GmbH, Gauting, Germany) and Sanger sequenced (LGC Genomics GmbH, Berlin, Germany). Experiments were carried out in duplicates. Fluorescence immuno-labeling of SM1-MSI cells in biofilms For the production of hamus-specific antibodies, hami filaments were released from the cells as follows. Biofilm samples were incubated in KPH buffer (NaCl 0.7 mM, MgCl 2 0.1 mM, CaSO 4 1.6 mM, HEPES 1.0 mM, supplemented with 0.1% SDS (v/v)) for 25 min and periodically vortexed, causing SM1 euryarchaeal cells to dissolve completely. The resulting suspension was centrifuged (30 min, 5,500 × g , 20 °C) to remove larger precipitates and the supernatant containing hami was ultracentrifuged (1 h, 92,387.1 × g , Beckman OPTIMA LE 80 K, 70.1 Ti-Rotor, 4 °C). The pellet was re-suspended in 2 ml of KPH buffer and applied on a sucrose-gradient (10–70% sucrose (w/v) in sterile KPH) and centrifuged for 17 h (309,000 × g , Beckman OPTIMA LE 80 K, SW 60 Rotor, 4 °C). The band appearing in the lower third of the tube was removed using a sterile syringe. After confirming the presence of hami via transmission electron microscopy (see below) the sample was sent to Davids biotechnology (Regensburg, Germany) for antibody production. A chicken was pre-immunized with the hami-fraction (0.22 mg/ml) three times over the course of 21 days. 28 days after the first immunization, eggs were collected and the IgG fraction (‘anti-hamus’; 15.1 mg/ml in 0.02% sodium-azide) was harvested. For immuno-staining, collected biofilms were fixed with paraformaldehyde (5% (v/v)) at room temperature (1 h) and washed three times with 1x PBS (phosphate buffered saline). Afterwards, fixed cells were incubated at 30 °C in PBST (PBS including Tween20 0.05% (v/v) with 0.1% SDS (v/v)) for 15 min, followed by a centrifugation step (15 min, 14,500 × g , 20 °C). The first primary antibody, anti-Anabaena FtsZ [60] (AS07217, Agrisera; dilution 1:200) was added and incubated at 30 °C for 2 h. Cells were centrifuged, followed by incubation in PBST (+0.1% SDS (v/v)) for 15 min and another centrifugation step. After incubation for 1 h with the conjugated goat anti-rabbit IgG (dilution 1:200), the cells were washed twice with PBST (+0.1% SDS (v/v)), spread within a well of a gelatine-coated slide (P. Marienfeld KG, Lauda-Koenigshofen, Germany) and fixed via air-drying. After incubation with 16 μl of PBST (+0.1% SDS (v/v)) at 37 °C, the PBST buffer was replaced with 16 μl PBST buffer containing the anti-hamus IgG (dilution 1:2,000) and the cells were labeled at 37 °C for 1 h. Subsequently, the slide was washed 15 min in PBST (+0.1% SDS (v/v)), rinsed with H 2 O and air dried. The second antibody (goat anti-chicken, Cy3-labeled; 0.64 mg/ml, dilution 1:500) was added and incubated at 37 °C for 1 h. After washing two times with PBST (+0.1% SDS (v/v)), the slide was rinsed with H 2 O, DAPI stained and analyzed using fluorescence microscopy (Olympus (BX53F, Hamburg, Germany) with epifluorescence equipment and imaging software cellSens). Transmission and scanning electron microscopy of MSI biofilms For TEM, fresh, unfixed biofilm pieces were deposited on a carbon-coated copper grid and negatively stained with 2% (w/v) uranyl acetate, pH 4.5 or 2.0% (w/v) phosphotungstic acid (PTA), pH 7.0. In a second approach, biofilms were treated with 1% SDS (w/v) for 30 min, causing destruction of the cell wall and thus a release of cell appendages. These samples were examined using a CM12 transmission electron microscope (FEI, Eindhoven, The Netherlands) operated at 120 keV. All images were digitally recorded using a slow-scan charge-coupled device camera that was connected to a computer with TVIPS software (TVIPS GmbH, Gauting, Germany). For conventional fixation, freshly taken biofilms were fixed in original spring water including 0.1% (w/v) glutardialdehyde. Samples were rinsed several times in fixative buffer and postfixed at room temperature for 1 h with 1% (w/v) osmium tetroxide. After two washing steps in water, the cells were stained for 30 min with 1% (w/v) uranyl acetate in 20% (v/v) acetone. Dehydration was performed by a graded acetone series. Samples were then infiltrated and embedded in Spurr’s low-viscosity resin. For high-pressure freezing experiment samples were frozen either with a Leica HPM100 (Leica Microsystems GmbH, Wetzlar, Germany, Fig. 5 ) or a Wohlwend HPF Compact 02 (Engineering Office M-Wohlwend GmbH, Sennwald, Switzerland; Fig. 4 ). In the first case aluminum platelets were used which were filled with one piece of biofilm. Freeze substitution was performed in acetone with 2% (w/v) osmium tetroxide and 0.2% (w/v) uranyl acetate, including 5% (v/v) water. After embedding the samples in Spurr’s low-viscosity resin, ultrathin sections were cut with a diamond knife and mounted onto uncoated copper grids. The sections were poststained with aqueous lead citrate (100 mM, pH 13.0). Transmission electron micrographs of samples prepared this way were taken with an EM 912 electron microscope (Zeiss) equipped with an integrated OMEGA energy filter operated at 80 kV in the zero loss mode. For SEM, drops of the sample were placed onto a glass slide, covered with a coverslip, and rapidly frozen with liquid nitrogen. The coverslip was removed with a razor blade and the glass slide was immediately fixed with 2.5% (w/v) glutaraldehyde in 10 mM cacodylate buffer (pH 7.0), postfixed with 1% (w/v) osmium tetroxide in fixative buffer, dehydrated in a graded series of acetone solutions, and critical-point dried after transfer to liquid CO 2 . Specimens were mounted on stubs, coated with 3 nm platinum using a magnetron sputter coater, and examined with a Zeiss Auriga scanning electron microscope operated at 1–2 kV. When using the Wohlwend HPF Compact 02, biofilm aggregates were placed in the centre of 3 mm gold carriers and high pressure frozen with a and subsequently freeze substituted in an automatic EM AFS 2 unit (Leica Microsystems GmbH, Wetzlar, Germany). The substitution medium consisted of acetone in combination with 0.2% (w/v) osmium tetroxide, 0.25% (w/v) uranyl acetate and 5% (v/v) water. The substitution program including washing steps and the following epon embedding, thin sectioning and post staining was carried out as described previously [61] . For these samples, microscopy was performed on a JEOL JEM-2100 (JEOL, Tokyo, Japan) also operated at 120 kV and equipped with a 2 k × 2 k fast scan CCD camera F214 combined with EM Menu4 (TVIPS GmbH, Gauting, Gemany). FIB-SEM tomography of MSI biofilms The focused ion beam FIB block face serial sectioning was performed using a Zeiss-Auriga workstation. The focused ion beam consisted of Ga + ions accelerated by a voltage of 30 kV. In the cut-and-view mode, sections ranging in thickness between 5 nm and 10 nm (dependent on the magnification) were produced with the FIB and field emission scanning electron microscopy (FESEM) images, which were recorded at 1.5 kV using the in-lens energy selective backscattered (EsB) detector set to −1,200 V. Specimens were tilted to an angle of 54°; images were tilt corrected for undistorted surface view. Lipid extraction and HPLC-MS analysis from biofilms Total lipid extracts (TLEs) were obtained from samples of the biofilm from MSI site using a modified Bligh and Dyer protocol [62] , after adding an internal standard (phosphatidylcholine C21:0/21:0) and 3 g of combusted sea sand. Approximately 10 8 to 10 9 cells were subjected to extraction. The obtained TLEs were stored at −20 °C and analysis of IPLs was performed by high-performance liquid chromatography electrospray ionization mass spectrometry (HPLC-ESI-MS). Separation of IPLs was achieved on a Dionex Ultimate 3000 UHPLC equipped with a Waters Acquity UPLC BEH Amide column (150 × 2.1 mm, 1.8 μm particle size). Chromatographic conditions, according to a previously published method [63] , were as follows: constant flow rate of 0.4 ml/min with eluent A (75% acetonitrile; 25% DCM; 0.01% formic acid; 0.01% ammonium hydroxide solution (NH 3 aq)) and eluent B (50% MeOH; 50% Milli-Q water; 0.4% formic acid; 0.4% NH 3 aq). Under a constant flow, the HPLC routine applied: 99% A and 1% B for 2.5 min, increasing to 5% B at 4 min, followed by a linear gradient to 25% B at 22.5 min and then to 40% B at 26.5 min. Thereafter a 1 min washing step with 40% B followed and afterwards reset to the initial conditions for 8 min to achieve column re-equilibration. Compound detection was conducted on a Bruker maXis Ultra-High Resolution qToF-MS, equipped with an ESI interface. IPLs were measured in positive ionization mode, while scanning a mass-to-charge (m/z) range of 150–2,000, with automated data-dependent MS/MS fragmentation of base peak ions. Compound identification was achieved by monitoring exact masses of possible parent ions (present mainly as H + and NH 4 + adducts) in combination with characteristic fragmentation patterns [62] , [64] . The reported relative distribution of microbial lipids is based on the peak areas of the respective molecular ions without differentiating for potential differences in response factors; the data should therefore be viewed as semi-quantitative. Stable carbon isotope analyses at MSI site Stable carbon isotopic (δ 13 C) composition of gases and lipids was obtained from groundwater samples and SM1 biofilm biomass. The δ 13 C values of CO 2 and CH 4 were measured from the headspace of groundwater samples (taken anaerobically and frozen on dry ice at MSI site by gas chromatography (GC) coupled to isotope-ratio mass spectrometry (irMS) (Trace GC ultra+DeltaPlus XP irMS, ThermoFinnigan). Given the dominance of glycolipids among both archaeal and bacterial lipids, TLEs were acid hydrolyzed (2.5% HCl in methanol) and derivatized with N,O-bis(trimethylsilyl)trifluoroacetamide in pyridine prior to GC-irMS (Trace GC Ultra coupled to a GC-IsoLink/ConFlow IV interface and a Delta V Plus irMS; all from Thermo Scientific). δ 13 C values of lipids were corrected for additional carbon introduced during derivatization. The δ 13 C values are expressed versus Vienna PeeDee Belemnite (VPDB). Measurements of gases and lipids in GC-irMS were performed at least in duplicate and the analytical error was <0.5‰. NanoSIMS, Raman spectroscopy, and conductivity experiments These were performed on MSI biofilm samples as described in the Supplementary Methods . Analysis of diversity and distribution of the SM1 group This is presented in the Supplementary Methods , and all accession codes are provided in Supplementary Table 6 . How to cite this article : Probst, A. J. et al . Biology of a widespread uncultivated archaeon that contributes to carbon fixation in the subsurface. Nat. Commun. 5:5497 doi: 10.1038/ncomms6497 (2014). Accession codes : The annotated SM1-MSI genome from the Mühlbacher Schwefelqulle (including the raw Illumina and 454 data) was deposited in the European Nucleotide Archive (study with accession code PRJEB6121 ). Raw Illumina data of the 3.0 filter sample from Crystal Geyser have been deposited in the Sequence Read Archive under accession code SRR1534154 . 16S rRNA gene sequences collected from various springs in Bavaria have been deposited in the NCBI Genbank database under accession codes KJ566428 to KJ566522 .